Epidermal cells help coordinate leukocyte migration during inflammation through fatty acid-fuelled matrix metalloproteinase production In addition to satisfying the metabolic demands of cells, mitochondrial metabolism helps regulate immune cell function. To date, such cell-intrinsic metabolic-immunologic cross-talk has only been described operating in cells of the immune system. Here we show that epidermal cells utilize fatty acid β-oxidation to fuel their contribution to the immune response during cutaneous inflammation. By live imaging metabolic and immunological processes within intact zebrafish embryos during cutaneous inflammation, we uncover a mechanism where elevated β-oxidation-fuelled mitochondria-derived reactive oxygen species within epidermal cells helps guide matrix metalloproteinase-driven leukocyte recruitment. This mechanism requires the activity of a zebrafish homologue of the mammalian mitochondrial enzyme, Immunoresponsive gene 1. This study describes the first example of metabolic reprogramming operating within a non-immune cell type to help control its contribution to the immune response. Targeting of this metabolic–immunologic interface within keratinocytes may prove useful in treating inflammatory dermatoses. Investigating how metabolism shapes the immune response is gaining significant attention due to the emerging connection between metabolic and inflammatory processes. Fuelled by the obesity epidemic, this new field of immunometabolism is underpinned by observations that inflammation is a hallmark of many chronic metabolic conditions [1] , [2] . In addition to the activation of immune cells within metabolic tissues, functional heterogeneity of immune cells can be regulated, on many levels, by cell-intrinsic metabolic reprogramming [3] , [4] , [5] . Whether non-immune cells also contribute to the immune response through coupling metabolism and immune function is, at present, unclear. Mitochondria are emerging as key organizers of innate immune cell function [6] . One mechanism through which mitochondria can influence immune cell activity is through elevated production of mitochondrial reactive oxygen species (mROS). Although a major source of cellular ROS, mROS have traditionally been regarded as insignificant by-products of oxidative phosphorylation (OXPHOS). More recent studies have identified inflammation-responsive mechanisms that elevate mROS and shown that mROS can have direct antibacterial activity and influence the expression of immune-response genes [6] , [7] , [8] . Whether non-immune cells also couple metabolic and inflammatory processes during their contribution to the immune response is unclear. In addition to providing a physical barrier protecting the host from its environment, the skin is a critical component of the immune system [9] . The immune response during cutaneous inflammation relies on finely tuned communication between immune cell subsets and non-immune cells such as epidermal keratinocytes [10] . Dysregulation of this communication can lead to inadequate or persistent inflammation that characterizes many inflammatory dermatoses [11] . In response to infection or injury keratinocytes produce matrix metalloproteinases (MMPs), a family of enzymes that collectively degrade all components of the extracellular matrix (ECM) [12] , [13] . The recruitment of leukocytes from the bloodstream and their migration through the ECM to sites of inflammation is, in part, dependent upon MMP activity. It has been suggested that keratinocyte-derived MMP9 production facilitates migration of leukocytes into the inflamed epidermis during cutaneous inflammation [13] . Both the expression and activity of MMPs has been shown to be directly regulated by mROS [14] . Furthermore, tumour necrosis factor alpha (TNF-α)-driven MMP9 expression within human keratinocytes is ROS-dependent [15] . Collectively, these data suggest mROS production within keratinocytes may promote leukocyte migration through regulation of MMP activity. These results also imply a possible connection between the metabolic process of OXPHOS within epidermal cells and leukocyte recruitment. The zebrafish is a well-established model to investigate innate immune cell function [16] . By 2 days post fertilization (dpf) zebrafish larvae are populated with neutrophil and macrophage lineages. Live imaging these innate immune cells within transgenic reporter lines has revealed remarkable conservation of function with their mammalian equivalents [17] , [18] , [19] , [20] . Live imaging analyses have also given unique insights into leukocyte behaviour during wound-associated cutaneous inflammation [21] , [22] , [23] , [24] . In contrast to the mammalian epidermis that consists of proliferating and differentiated keratinocytes within several strata, the epidermis of embryonic/larval zebrafish is relatively simple consisting of an outermost enveloping and inner epidermal basal layer [25] , [26] . Despite this simple architecture, functional similarities exist between the zebrafish and mammalian epidermis, supporting the use of zebrafish as a model of skin diseases [26] , [27] , [28] . Exploiting the live imaging potential of the zebrafish system, previous work in our group has revealed activated macrophages utilize β-oxidation of fatty acids to fuel OXPHOS-coupled mROS that contributes to macrophage effector function [7] . This metabolic reprogramming of macrophages requires a mitochondrial enzyme encoded by immunoresponsive gene 1 ( irg1 ), a vertebrate homologue of a bacterial enzyme necessary for fatty acid metabolism [29] . Zebrafish possess 2 IRG1 homologues, irg1 and irg1-like ( irg1l ), most likely the result of a duplication event. A recent study has suggested a function for Irg1l during cutaneous inflammation [30] . We predicted that Irg1l may couple metabolic and immunological processes, similar to its paralog Irg1. Using the zebrafish system to explore the function of Irg1l, we uncover a new Irg1l-dependent signalling pathway that connects metabolic and inflammatory processes within epidermal cells during inflammation. We demonstrate expression of irg1l within epidermal cells in response to live bacterial infection and wound-induced inflammation, where it contributes to leukocyte recruitment. In response to bacterial infection, epidermal cells enhance their production of mROS in a process dependent on Irg1l and fuelled by fatty acid β-oxidation. We further show that Irg1l and β-oxidation are necessary for infection- and wound-responsive mmp9 expression within epidermal cells that demonstrate elevated mitochondrial uptake of fatty acids. Finally, we demonstrate elevated abundance of IRG1 within mitochondria of keratinocytes in a mouse model of cutanous inflammation (atopic dermatitis) supporting the translation of our zebrafish findings to a mammalian setting. We propose a new mechanism where Irg1l-dependent β-oxidation-fuelled mROS production within epidermal cells contributes to MMP-9-driven leukocyte migration during inflammation. For the first time, this study connects inflammation-driven changes in epidermal cell metabolism with their contribution to the immune response. This suggests that metabolic reprogramming, as a mechanism to help orchestrate the immune response, is not restricted to immune cells. irg1l is expressed by epidermal cells following infection We first identified zebrafish Irg1l (a homologue of mammalian IRG1) as a gene upregulated in response to live Salmonella enterica serovar Typhimurium (hereafter referred to as Salmonella ) infection using the GeneChip Zebrafish Genome Array (Affymetrix) ( Fig. 1a ), consistent with a previous study [30] . Quantitative (q) PCR analysis of irg1l expression following Salmonella infection (~\n600 colony-forming units (cfu) injected into the hindbrain ventricle of 2 dpf larvae) revealed elevated expression from 1 h post injection (hpi), when compared with PBS-injected controls ( Fig. 1b ). Infection-responsive expression of irg1l peaked at 1 day post injection (dpi) before returning to ‘steady-state’ levels by 3 dpi ( Fig. 1b ). Throughout this study, unless otherwise stated, an infection dose of 600 cfu of Salmonella was injected into the hindbrain ventricle of 2 dpf larvae to stimulate an antibacterial immune response. When compared with PBS-injected controls, Salmonella -injected larvae (2 hpi) possessed infection-responsive irg1l expression within cells covering the infection site as well as within nasal and neuromast epithelial cells ( Fig. 1c,d ). Constitutive expression of irg1l was detected within epithelial cells of the oropharyngeal region and cloaca ( Fig. 1c ). Injection of E. coli lipopolysaccharide (LPS) also stimulated similar early irg1l expression ( Supplementary Fig. 1 ). Of note, LPS-stimulated irg1l expression did not persist as long as that induced by live Salmonella injection ( Supplementary Fig. 1 ). By 1 dpi, infection-responsive expression of irg1l became largely restricted to neuromasts of the developing lateral line system ( Supplementary Fig. 2a,b ). Some infected larvae also possessed irg1l expression within the intestine and pronephric tubules ( Supplementary Fig. 2c,d ). In light of the well-recognized contribution that the epidermis/skin provides to a functional immune system, we investigated the role of Irg1l within the epidermis. Expression analysis revealed that epithelial cells with infection-responsive irg1l expression, surrounding the infection site, were also positive for the epidermal marker keratin 4 ( krt4 ), as detected at 4 hpi ( Fig. 1e ). To visualize epidermal irg1l expression with respect to injected bacteria, we utilized GFP-expressing Salmonella (hereafter referred to as Sal-GFP) [31] . Injected Sal-GFP were observed in close proximity to (but never within) overlying irg1l + epidermal cells ( Fig. 1f ). Transcriptome profiling has previously demonstrated expression of irg1l to be elevated in response to both intravenous injection of, and immersion in, the natural fish pathogen Edwardsiella tarda [30] . In contrast to this study, we were not able to detect epidermal expression of irg1l following immersion in live Salmonella or LPS, as detected by whole-mount in situ hybridization (WMISH) analysis ( Supplementary Fig. 2e–h ). This suggests, in our infection model, host-derived endogenous signals contribute to infection-responsive expression of irg1l within epidermal cells. 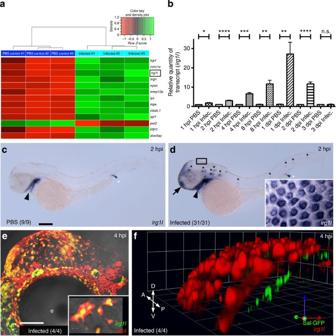Figure 1: Irg1l is expressed withinkrt4+epidermal cells followingSalmonellainfection. (a) Heat map illustrating differentially abundant mRNAs between infected (hindbrainSalmonella-injected) and PBS-injected larvae (in biological triplicate). (b) qPCR analysis ofirg1lexpression following infection, measured at 1 hpi, 2 hpi, 4 hpi, 8 hpi, 1 dpi, 2 dpi and 3 dpi, relative to PBS-injected controls (mean±s.d.;n=3 biological replicates, ~\n50 larvae per group). (c,d) Expression analysis ofirg1lwithin PBS control and infected larvae at 2 hpi, respectively (n=2 separate infection experiments, lateral views, anterior to left). Inset, magnified dorsal view of boxed region ind. Arrowhead and white asterisk mark constitutiveirg1lexpression within oropharyngeal region and cloaca, respectively. Arrow and black asterisks mark infection-responsiveirg1lexpression within nasal and neuromast epithelium, respectively. (e) Expression ofirg1lwithinkrt4+epidermal cells covering the head following infection, as detected at 4 hpi (lateral view, anterior to left). Inset, magnified view of individual cells co-expressingirg1landkrt4. (f) 3D transverse view demonstratingirg1lexpression within epidermal cells of the midbrain/hindbrain region overlying injected GFP-expressingSalmonella, at 4 hpi. Numbers represent frequencies of larvae with displayed phenotypes. Scale bars, 100 μm inc; 50 μm ine. Statistical significance determined using a Student’st-test. *P-value <0.05; **P-value <0.01; ***P-value<0.001; ****P-value <0.0001; n.s., not significant; e, eye; A, anterior; P, posterior; D, dorsal; V, ventral. Figure 1: Irg1l is expressed within krt4 + epidermal cells following Salmonella infection. ( a ) Heat map illustrating differentially abundant mRNAs between infected (hindbrain Salmonella -injected) and PBS-injected larvae (in biological triplicate). ( b ) qPCR analysis of irg1l expression following infection, measured at 1 hpi, 2 hpi, 4 hpi, 8 hpi, 1 dpi, 2 dpi and 3 dpi, relative to PBS-injected controls (mean±s.d. ; n =3 biological replicates, ~\n50 larvae per group). ( c , d ) Expression analysis of irg1l within PBS control and infected larvae at 2 hpi, respectively ( n =2 separate infection experiments, lateral views, anterior to left). Inset, magnified dorsal view of boxed region in d . Arrowhead and white asterisk mark constitutive irg1l expression within oropharyngeal region and cloaca, respectively. Arrow and black asterisks mark infection-responsive irg1l expression within nasal and neuromast epithelium, respectively. ( e ) Expression of irg1l within krt4 + epidermal cells covering the head following infection, as detected at 4 hpi (lateral view, anterior to left). Inset, magnified view of individual cells co-expressing irg1l and krt4 . ( f ) 3D transverse view demonstrating irg1l expression within epidermal cells of the midbrain/hindbrain region overlying injected GFP-expressing Salmonella , at 4 hpi. Numbers represent frequencies of larvae with displayed phenotypes. Scale bars, 100 μm in c ; 50 μm in e . Statistical significance determined using a Student’s t -test. * P -value <0.05; ** P -value <0.01; *** P -value<0.001; **** P -value <0.0001; n.s., not significant; e, eye; A, anterior; P, posterior; D, dorsal; V, ventral. Full size image These results demonstrate that irg1l is rapidly expressed within epidermal cells in response to bacterial infection. Macrophages are required for epidermal irg1l expression We have previously shown macrophages respond, and functionally contribute, to the immune response in our hindbrain infection model [31] . We next investigated whether host-derived signals necessary for epidermal irg1l expression were macrophage-dependent. We took advantage of the ability of spleen focus-forming virus proviral integration oncogene (Spi1)- and granulocyte colony stimulating factor receptor (Gcsfr)-targeting morpholino oligonucleotides (MOs) to deplete larvae of both the macrophage and neutrophil lineages, to first assess the myeloid-lineage contribution to infection-responsive epidermal irg1l expression [31] , [32] . Larvae depleted of both Spi1 and Gcsfr demonstrated a decrease in epidermal irg1l expression following infection ( Fig. 2a ). To differentiate whether this myeloid-lineage contribution to infection-responsive irg1l expression was at the level of the macrophage or neutrophil, we next evaluated irg1l expression within interferon regulatory factor 8 (Irf8)-depleted larvae following infection. The transcription factor Irf8 has been shown to regulate macrophage versus neutrophil lineage commitment such that Irf8-depleted larvae possess an expanded neutrophil compartment and depleted numbers of macrophages [33] . Similar to larvae depleted of both Spi1 and Gcsfr, Irf8-depleted larvae demonstrated a decrease in epidermal irg1l expression following infection ( Fig. 2a ). These results suggest macrophages contribute to infection-responsive epidermal irg1l expression. To visualize macrophages in relation to injected bacteria and epidermal irg1l expression, we exploited the macrophage-lineage marking Tg ( mpeg1:Gal4/UAS:Kaede ) reporter line [17] . Analysis of irg1l expression within Tg ( mpeg1:Gal4/UAS:Kaede ) larvae following Sal-GFP injection showed macrophage expressed 1 (Mpeg1) + macrophages and bacteria in close proximity to overlying irg1l + epidermal cells, as assessed at 4 hpi ( Fig. 2b ). Live imaging infected Tg ( mpeg1:mCherry ) [17] larvae demonstrated that these macrophages were highly phagocytic toward the injected Sal-GFP ( Fig. 2c ). 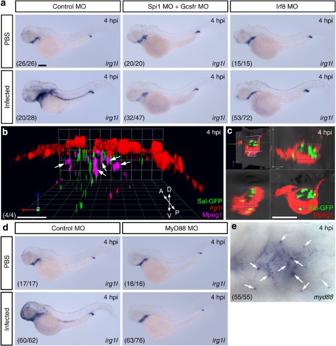Figure 2: Infection-responsive epidermal expression ofirg1lis dependent upon macrophages and Myd88. (a) Expression ofirg1lwithin control MO-, Spi1 MO + Gcsfr MO- and Irf8 MO-injected larvae following PBS andSalmonellainjection, as detected at 4 hpi (n=2 separate infection experiments, lateral views, anterior to left). Remainder of infected control MO-injected (8/28), Spi1/Gcsfr- (15/47) and Irf8- (19/72) depleted larvae displayed weak epidermalirg1lexpression. (b) 3D transverse view of midbrain/hindbrain region ofTg(mpeg1:Gal4/UAS:Kaede), larvae demonstratingirg1l-expressing epidermal cells overlying Sal-GFP and Mpeg1+macrophages (white arrows) following infection, as detected by immunofluorescence at 4 hpi. (c) Live imaging Sal-GFP within Mpeg1+macrophages, at 4 hpi, within midbrain/hindbrain region ofTg(mpeg1:mCherry) larvae following infection. (d) Expression ofirg1lwithin control MO-injected and MyD88-depleted larvae following PBS andSalmonellainjection, as detected at 4 hpi (n=3 separate infection experiments, lateral views, anterior to left). Remainder of infected control MO-injected (2/62) and MyD88-depleted (13/76) larvae displayed weak epidermalirg1lexpression. (e) Expression ofmyd88within the midbrain/hindbrain region, at 4 hpi, following infection (n=3 separate infection experiments, dorsal view, anterior to left). Arrows mark presumptivemyd88-expressing macrophages. Numbers represent frequencies of larvae with displayed phenotypes. Scale bars, 100 μm ina; 50 μm inb; 10 μm inc. A, anterior; P, posterior; D, dorsal; V, ventral. Figure 2: Infection-responsive epidermal expression of irg1l is dependent upon macrophages and Myd88. ( a ) Expression of irg1l within control MO-, Spi1 MO + Gcsfr MO- and Irf8 MO-injected larvae following PBS and Salmonella injection, as detected at 4 hpi ( n =2 separate infection experiments, lateral views, anterior to left). Remainder of infected control MO-injected (8/28), Spi1/Gcsfr- (15/47) and Irf8- (19/72) depleted larvae displayed weak epidermal irg1l expression. ( b ) 3D transverse view of midbrain/hindbrain region of Tg ( mpeg1:Gal4/UAS:Kaede ), larvae demonstrating irg1l -expressing epidermal cells overlying Sal-GFP and Mpeg1 + macrophages (white arrows) following infection, as detected by immunofluorescence at 4 hpi. ( c ) Live imaging Sal-GFP within Mpeg1 + macrophages, at 4 hpi, within midbrain/hindbrain region of Tg ( mpeg1:mCherry ) larvae following infection. ( d ) Expression of irg1l within control MO-injected and MyD88-depleted larvae following PBS and Salmonella injection, as detected at 4 hpi ( n =3 separate infection experiments, lateral views, anterior to left). Remainder of infected control MO-injected (2/62) and MyD88-depleted (13/76) larvae displayed weak epidermal irg1l expression. ( e ) Expression of myd88 within the midbrain/hindbrain region, at 4 hpi, following infection ( n =3 separate infection experiments, dorsal view, anterior to left). Arrows mark presumptive myd88 -expressing macrophages. Numbers represent frequencies of larvae with displayed phenotypes. Scale bars, 100 μm in a ; 50 μm in b ; 10 μm in c . A, anterior; P, posterior; D, dorsal; V, ventral. Full size image A well-characterized mechanism through which innate immune cells detect bacteria is via the Toll-like receptor (TLR) class of pattern recognition receptors [34] . Cell surface and intracellular TLRs detect specific pathogen-associated molecular patterns, stimulating signalling cascades that couple pathogen detection to downstream immune cell functions, including cytokine production. TLR signalling is largely dependent on the adaptor molecule myeloid differentiation primary response gene 88 (MYD88). We have previously shown that innate immune cells in zebrafish express TLR adaptor molecules, including myd88 (ref. 18 ). In addition, zebrafish MyD88 has been demonstrated to contribute to pathogen clearance following infection [35] . To assess whether MyD88-dependent TLR signalling is required for irg1l expression within epidermal cells following infection, we analysed irg1l expression within infected MyD88-depleted larvae. Epidermal expression of irg1l was not detected within infected MyD88-depleted larvae ( Fig. 2d ). Analysis of myd88 expression within infected larvae revealed expression within putative macrophages in the midbrain/hindbrain region ( Fig. 2e ). Of note, expression was not detected within the overlying epidermis. These results suggest infection-responsive expression of irg1l within the epidermis requires macrophage detection of bacteria through a MyD88-dependent mechanism. GC signalling suppresses epidermal irg1l expression Glucocorticoids (GCs) are a class of steroid hormone that largely suppress the immune response. Through binding the glucocorticoid receptor (GR), GCs upregulate anti-inflammatory, while repressing pro-inflammatory, gene expression. GCs have been shown to possess conserved anti-inflammatory activity in larval zebrafish ( Supplementary Fig. 3a–c ) [36] . We next investigated whether the infection-responsive expression of irg1l within epidermal cells was sensitive to the anti-inflammatory activity of GC/GR signalling. To assess the effect of GCs on epidermal irg1l expression we co-injected Salmonella with dexamethasone, hydrocortisone and prednisolone and analysed irg1l expression at 4 hpi. In contrast to Salmonella alone, epidermal irg1l expression was not detected in co-injected larvae ( Fig. 3a ), suggesting GCs suppress infection-responsive expression of irg1l within epidermal cells. To evaluate the requirement for GR signalling during GC-mediated irg1l suppression, we co-injected Salmonella with the GR antagonist RU-486 and infected larvae depleted of the zebrafish ortholog of nuclear receptor subfamily 3, group C, member 1 (NR3C1) (encoding the GR), then assessed irg1l expression. When compared with control MO-injected infected larvae, RU-486-treated and Nr3c1-depleted larvae demonstrated elevated infection-responsive epidermal irg1l expression ( Fig. 3b ). In zebrafish, endogenous GCs are produced by the inter-renal tissue, which functions as an adrenal gland-equivalent. Inter-renal tissue and its steroidogenic activity can be ablated through knockdown of nuclear receptor subfamily 5, group A, member 1a (Nr5a1a) ( Supplementary Fig. 3d,e ) [37] . A similar increase in epidermal irg1l expression following infection was observed within larvae depleted of Nr5a1a ( Supplementary Fig. 3f ). Immunofluorescence detection of Nr3c1 within infected larvae revealed Nr3c1 protein localized to Mpeg1 + macrophages within, and irg1l -expressing epidermal cells overlying, the midbrain/hindbrain infection region ( Fig. 3c,d ). The greater sensitivity of this tyramide signal amplification-based fluorescence detection method revealed irg1l expression extended throughout the trunk within Nr3c1 + epidermal cells ( Supplementary Fig. 4 ). Of note, Nr3c1 also colocalized with other irg1l -expressing epithelial tissues including the neuromasts, cloaca, nasal epithelium and the oropharngeal region ( Supplementary Fig. 4 ). 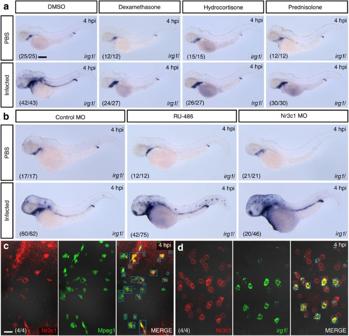Figure 3: GC/GR signalling suppresses infection-responsive expression ofirg1lin epidermal cells. (a) Expression ofirg1lwithin PBS control and infected larvae following DMSO, dexamethasone, hydrocortisone or prednisolone treatments, as detected at 4 hpi (n=2 separate infection experiments, lateral views, anterior to left). Remainder of infected DMSO- (1/43), dexamethasone- (3/27) and hydrocortisone-treated (1/27) larvae displayed weak epidermalirg1lexpression. (b) Expression ofirg1lwithin control MO-injected, RU-486-treated and Nr3c1-depleted larvae following PBS control andSalmonellainjection, as detected at 4 hpi (n=2 separate infection experiments, lateral views, anterior to left). Remainder of infected control MO-injected larvae (2/62) possessed weak epidermalirg1lexpression. Remainder of infected RU-486-treated (33/75) and Nr3c1-depleted (26/46) larvae displayedirg1lexpression similar to that shown for control MO-injected/infected. (c) Immunofluorescence detection of Nr3c1 within Mpeg1+macrophages, at 4 hpi, within the midbrain/hindbrain region ofTg(mpeg1:EGFP) larvae following infection. (d) Immunofluorescence detection of Nr3c1 withinirg1l-expressing epidermal cells, at 4 hpi, overlying the midbrain/hindbrain infection region. Boxes mark colocalized signal. Numbers represent frequencies of larvae with displayed phenotypes. Scale bars, 100 μm ina; 20 μm inc. Figure 3: GC/GR signalling suppresses infection-responsive expression of irg1l in epidermal cells. ( a ) Expression of irg1l within PBS control and infected larvae following DMSO, dexamethasone, hydrocortisone or prednisolone treatments, as detected at 4 hpi ( n =2 separate infection experiments, lateral views, anterior to left). Remainder of infected DMSO- (1/43), dexamethasone- (3/27) and hydrocortisone-treated (1/27) larvae displayed weak epidermal irg1l expression. ( b ) Expression of irg1l within control MO-injected, RU-486-treated and Nr3c1-depleted larvae following PBS control and Salmonella injection, as detected at 4 hpi ( n =2 separate infection experiments, lateral views, anterior to left). Remainder of infected control MO-injected larvae (2/62) possessed weak epidermal irg1l expression. Remainder of infected RU-486-treated (33/75) and Nr3c1-depleted (26/46) larvae displayed irg1l expression similar to that shown for control MO-injected/infected. ( c ) Immunofluorescence detection of Nr3c1 within Mpeg1 + macrophages, at 4 hpi, within the midbrain/hindbrain region of Tg ( mpeg1:EGFP ) larvae following infection. ( d ) Immunofluorescence detection of Nr3c1 within irg1l -expressing epidermal cells, at 4 hpi, overlying the midbrain/hindbrain infection region. Boxes mark colocalized signal. Numbers represent frequencies of larvae with displayed phenotypes. Scale bars, 100 μm in a ; 20 μm in c . Full size image Together, these results support a model where infection-responsive epidermal expression of irg1l is suppressed by the anti-inflammatory activity of GCs, most likely at the level of GR/Nr3c1 + macrophages and/or epidermal cells. Irg1l contributes to bacterial clearance To examine whether Irg1l contributes to the clearance of injected bacteria, we monitored bacterial persistence within Irg1l-depleted larvae infected with Sal-GFP. When compared with control MO-injected larvae, Irg1-depleted larvae demonstrated a significant increase in bacterial persistence, as assessed by live fluorescence microscopy ( Fig. 4a,b and Supplementary Fig. 5 ) and recovered bacteria ( Fig. 4c ). This defective bacterial clearance resulted in decreased survival post-infection ( Fig. 4d ). These data support a functional role for Irg1l during clearance of injected bacteria. 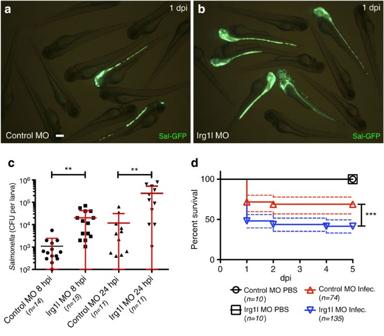Figure 4: Irg1l-depleted larvae demonstrate diminished bacterial clearance and reduced survival following infection. (a,b) Live imaging of control MO-injected and Irg1l-depleted larvae, respectively, following infection with GFP-labelledSalmonella, imaged at 1 dpi. (c) CFU counts of remaining GFP-labelledSalmonellawithin individual infected control MO-injected and Irg1l-depleted larvae quantified at 8 and 24 hpi (mean±s.d.;n=2 experiments). Statistical significance determined using a Student’st-test. (d) Kaplan–Meier survival graph demonstrating % survival of control MO-injected PBS-injected, Irg1l-depleted PBS-injected, control MO-injected infected and Irg1l-depleted infected larvae from 1 to 5 dpi. Significance of curve differences for control MO-infected and Irg1l-depleted infected groups calculated using Log-rank (Mantel–Cox) test,n=3 separate infection experiments (95% c.i. represented by dashed lines). Scale bar, 200 μm ina. **P-value<0.01; ***P-value<0.001. Figure 4: Irg1l-depleted larvae demonstrate diminished bacterial clearance and reduced survival following infection. ( a , b ) Live imaging of control MO-injected and Irg1l-depleted larvae, respectively, following infection with GFP-labelled Salmonella , imaged at 1 dpi. ( c ) CFU counts of remaining GFP-labelled Salmonella within individual infected control MO-injected and Irg1l-depleted larvae quantified at 8 and 24 hpi (mean±s.d. ; n =2 experiments). Statistical significance determined using a Student’s t -test. ( d ) Kaplan–Meier survival graph demonstrating % survival of control MO-injected PBS-injected, Irg1l-depleted PBS-injected, control MO-injected infected and Irg1l-depleted infected larvae from 1 to 5 dpi. Significance of curve differences for control MO-infected and Irg1l-depleted infected groups calculated using Log-rank (Mantel–Cox) test, n =3 separate infection experiments (95% c.i. represented by dashed lines). Scale bar, 200 μm in a . ** P -value<0.01; *** P -value<0.001. Full size image Irg1l contributes to epidermal mmp9 expression A feature of cutaneous inflammation associated with infection is the infiltration of innate immune cells, including monocytes/macrophages and neutrophils, into the dermis and epidermis. Central to the recruitment of leukocytes is the ECM-degrading activity of the MMP family of proteases [13] , [38] . Similar to mammals, bacterial infection can elevate the expression of mmp9 within the zebrafish larval epidermis ( Supplementary Fig. 6 ), where it contributes to macrophage recruitment [39] . We next investigated whether infection-responsive expression of irg1l within the epidermis contributes towards mmp9 expression and the recruitment of macrophages to the infection site. Fluorescent expression analysis confirmed irg1l and mmp9 expression colocalized within epidermal cells following infection ( Fig. 5a,b ). qPCR analysis of mmp9 expression within control MO-injected and Irg1l-depleted larvae at 1, 2 and 4 hpi revealed that Irg1l contributed to infection-responsive mmp9 expression ( Fig. 5c ). This result was supported when assessing mmp9 expression within infected control MO and Irg1l-depleted larvae ( Fig. 5d,e ). Irg1l-depleted Tg ( mpeg1:EGFP ) larvae also demonstrated reduced macrophage recruitment to the infection site, when compared with control MO-injected Tg ( mpeg1:EGFP ) larvae, despite maintaining unaltered (whole larvae) numbers of macrophages ( Fig. 5f,g and Supplementary Fig. 7 ). 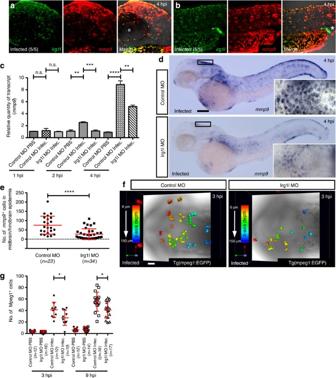Figure 5: Irg1l contributes to infection-responsivemmp9expression within epidermal cells and the recruitment of macrophages to the infection site. (a,b) Dual expression analysis ofirg1landmmp9within the head and trunk, respectively, following infection, as detected at 4 hpi (lateral views, anterior to left). White asterisk marksirg1l-expressing cloaca. (c) qPCR analysis ofmmp9expression within control MO-injected and Irg1l-depleted larvae following PBS control andSalmonellainjection, detected at 1, 2 and 4 hpi (mean±s.d.;n=3 biological replicates, ~\n50 larvae per group). (d) Expression ofmmp9within control MO-injected and Irg1l-depleted larvae following infection, as detected at 4 hpi (lateral views, anterior to left). Insets represent magnified dorsal views of boxed regions. (e) Quantification ofmmp9+epidermal cells covering the midbrain/hindbrain region of individual infected larvae as shown in d (mean±s.d.;n=2 separate infection experiments). (f) Detection of Mpeg1+cells, at 3 hpi, within the midbrain/hindbrain region of control MO-injected and Irg1l-depletedTg(mpeg1:EGFP) larvae following infection (dorsal views, anterior to left). Individual macrophages are pseudo-colored to reflectzaxis depth. (g) Quantification of Mpeg1+cells within the midbrain/hindbrain region of control MO-injected and Irg1l-depletedTg(mpeg1:EGFP) larvae (as detected inf), at 3 and 9 hpi, following PBS orSalmonellainjections (mean±s.d.;n=2 separate infection experiments). Scale bars, 50 μm ina; 100 μm ind; 20 μm inf. Statistical significance determined using a Student’st-test. *P-value<0.05; **P-value<0.01; ***P-value <0.001; ****P-value <0.0001; n.s., not significant; e, eye. Figure 5: Irg1l contributes to infection-responsive mmp9 expression within epidermal cells and the recruitment of macrophages to the infection site. ( a , b ) Dual expression analysis of irg1l and mmp9 within the head and trunk, respectively, following infection, as detected at 4 hpi (lateral views, anterior to left). White asterisk marks irg1l -expressing cloaca. ( c ) qPCR analysis of mmp9 expression within control MO-injected and Irg1l-depleted larvae following PBS control and Salmonella injection, detected at 1, 2 and 4 hpi (mean±s.d. ; n =3 biological replicates, ~\n50 larvae per group). ( d ) Expression of mmp9 within control MO-injected and Irg1l-depleted larvae following infection, as detected at 4 hpi (lateral views, anterior to left). Insets represent magnified dorsal views of boxed regions. ( e ) Quantification of mmp9 + epidermal cells covering the midbrain/hindbrain region of individual infected larvae as shown in d (mean±s.d. ; n =2 separate infection experiments). ( f ) Detection of Mpeg1 + cells, at 3 hpi, within the midbrain/hindbrain region of control MO-injected and Irg1l-depleted Tg ( mpeg1:EGFP ) larvae following infection (dorsal views, anterior to left). Individual macrophages are pseudo-colored to reflect z axis depth. ( g ) Quantification of Mpeg1 + cells within the midbrain/hindbrain region of control MO-injected and Irg1l-depleted Tg ( mpeg1:EGFP ) larvae (as detected in f ), at 3 and 9 hpi, following PBS or Salmonella injections (mean±s.d. ; n =2 separate infection experiments). Scale bars, 50 μm in a ; 100 μm in d ; 20 μm in f . Statistical significance determined using a Student’s t -test. * P -value<0.05; ** P -value<0.01; *** P -value <0.001; **** P -value <0.0001; n.s., not significant; e, eye. Full size image These results suggest that Irg1l contributes to the recruitment of macrophages to the infection site through regulating epidermal mmp9 expression. Irg1l regulates epidermal mmp9 expression following wounding In addition to infection, cutaneous inflammation associated with wound healing, allergy and/or trauma also requires the timely recruitment of specific leukocyte subsets. Employing a well-characterized tail transection model of acute wound-associated inflammation ( Fig. 6a ) [17] , [40] , we examined whether irg1l was expressed in response to wounding and, if so, whether it helped coordinate the inflammatory phase of wound healing. 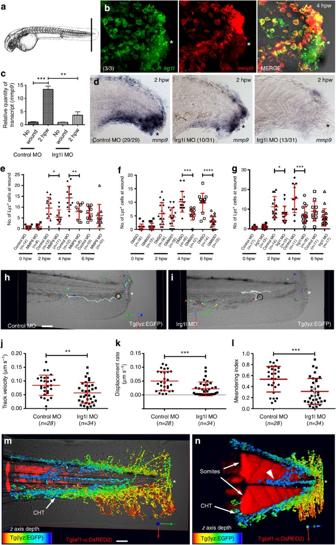Figure 6: Irg1l contributes to epidermalmmp9expression and the recruitment of neutrophils to wounded tissues. (a) Schematic of tail transection within 2 dpf larvae (all wounds were generated at the same anatomic location). (b) Expression ofirg1landmmp9within larvae at 4 h post wounding (hpw), magnified view of transected tail (lateral views, anterior to left). (c) qPCR analysis ofmmp9expression within control MO-injected and Irg1l-depleted larvae, relative to non-wounded controls, at 2 hpw (mean±s.d.;n=3 biological replicates, ~\n50 larvae per group). (d) Expression ofmmp9within control MO-injected and Irg1l-depleted larvae at 2 hpw (n=2 separate wounded cohorts, lateral views, anterior to left). Magnified views of transected tails revealing Irg1l-depleted larvae with reduced (10/31) and abolished (13/31) wound-inducedmmp9expression. Remainder of wounded Irg1l-depleted larvae (8/31) displayedmmp9expression similar to that shown for control MO-injected. (e–g) Quantification of Lyz+neutrophils within wounded control MO-injected and MMP9-depleted (e), DMSO- and GM6001-treated (f), and control MO-injected and Irg1l-depleted (g)Tg(lyz:EGFP) larvae at 0, 2, 4 and 6 hpw (mean±s.d.;n=2 separate wounded cohorts). Neutrophils quantified within wound region extending 100 μm from wound border. (h,i) Individual neutrophil tracks within wounded control MO-injected and Irg1l-depletedTg(lyz:EGFP) larvae, respectively (lateral views, anterior to left). Circles highlight tracked neutrophils at the end of tracks. (j–l) Track velocities, displacement rates and meandering indices, respectively, of individual neutrophil tracks, as detected inhandi(mean±s.d.;n=3 individual control MO-injected and Irg1l-depleted wounded larvae). (m) Neutrophil tracks within woundedTg(lyz:EGFP)/Tg(ef1-α:DsRED2) double transgenic larvae (from 15 h time-lapse experiment) with tracks pseudo-colored to reflectzaxis depth (colder colours represent tracks closer to viewer). Lateral view, anterior to left. (n) 3D transverse view ofmrevealing neutrophils migrating over surface of red-fluorescent somites (white arrowhead)en routeto wound. White and black asterisks mark wound border. Scale bars, 20 μm inb; 50 μm inhandm. Statistical significance determined using a Student’st-test. CHT, caudal hematopoietic tissue; *P-value <0.05; **P-value <0.01; ***P-value <0.001; ****P-value <0.0001. Figure 6: Irg1l contributes to epidermal mmp9 expression and the recruitment of neutrophils to wounded tissues. ( a ) Schematic of tail transection within 2 dpf larvae (all wounds were generated at the same anatomic location). ( b ) Expression of irg1l and mmp9 within larvae at 4 h post wounding (hpw), magnified view of transected tail (lateral views, anterior to left). ( c ) qPCR analysis of mmp9 expression within control MO-injected and Irg1l-depleted larvae, relative to non-wounded controls, at 2 hpw (mean±s.d. ; n =3 biological replicates, ~\n50 larvae per group). ( d ) Expression of mmp9 within control MO-injected and Irg1l-depleted larvae at 2 hpw ( n =2 separate wounded cohorts, lateral views, anterior to left). Magnified views of transected tails revealing Irg1l-depleted larvae with reduced (10/31) and abolished (13/31) wound-induced mmp9 expression. Remainder of wounded Irg1l-depleted larvae (8/31) displayed mmp9 expression similar to that shown for control MO-injected. ( e – g ) Quantification of Lyz + neutrophils within wounded control MO-injected and MMP9-depleted ( e ), DMSO- and GM6001-treated ( f ), and control MO-injected and Irg1l-depleted ( g ) Tg ( lyz:EGFP ) larvae at 0, 2, 4 and 6 hpw (mean±s.d. ; n =2 separate wounded cohorts). Neutrophils quantified within wound region extending 100 μm from wound border. ( h , i ) Individual neutrophil tracks within wounded control MO-injected and Irg1l-depleted Tg ( lyz:EGFP ) larvae, respectively (lateral views, anterior to left). Circles highlight tracked neutrophils at the end of tracks. ( j – l ) Track velocities, displacement rates and meandering indices, respectively, of individual neutrophil tracks, as detected in h and i (mean±s.d. ; n =3 individual control MO-injected and Irg1l-depleted wounded larvae). ( m ) Neutrophil tracks within wounded Tg ( lyz:EGFP )/ Tg ( ef1- α :DsRED2 ) double transgenic larvae (from 15 h time-lapse experiment) with tracks pseudo-colored to reflect z axis depth (colder colours represent tracks closer to viewer). Lateral view, anterior to left. ( n ) 3D transverse view of m revealing neutrophils migrating over surface of red-fluorescent somites (white arrowhead) en route to wound. White and black asterisks mark wound border. Scale bars, 20 μm in b ; 50 μm in h and m . Statistical significance determined using a Student’s t -test. CHT, caudal hematopoietic tissue; * P -value <0.05; ** P -value <0.01; *** P -value <0.001; **** P -value <0.0001. Full size image Similar to that induced by bacterial injection, irg1l was expressed within epidermal cells at the wound site by 1 hour post wounding (hpw) ( Supplementary Fig. 8a,b ). Expression analysis confirmed that irg1l -expressing epidermal cells also expressed mmp9 ( Fig. 6b ). Irg1l-depleted larvae demonstrated a reduction in wound-induced epidermal mmp9 expression, when compared with control larvae, suggesting Irg1l is required, at least in part, for wound-induced epidermal mmp9 expression ( Fig. 6c,d ). As ‘first responders’ during inflammation, neutrophils are the first leukocytes to arrive at wounded tissues. Live imaging of wounded transgenic zebrafish larvae possessing fluorescent neutrophils has provided unique insights into the migratory kinetics of these innate immune cells [23] , [24] , [41] . By live imaging Tg ( lyz:EGFP ) larvae we assessed whether Irg1l-regulated mmp9 expression contributed to the recruitment of lysozyme (Lyz) + neutrophils to wounded tissue. To first evaluate whether MMP9 contributes to neutrophil recruitment in our model, we assessed neutrophil recruitment to tail wounds within MMP9-depleted larvae and larvae treated with the pan-MMP inhibitor GM6001 (ref. 42 ). In contrast to control larvae, MMP9-depleted and GM6001-treated larvae possessed fewer neutrophils at the wound region ( Fig. 6e,f and Supplementary Fig. 9 ), despite maintaining typical (whole-larva) numbers of neutrophils ( Supplementary Fig. 10 ). A similar reduction was also observed within Irg1-depleted larvae ( Fig. 6g ), despite maintaining typical (whole-larvae) numbers of neutrophils ( Supplementary Fig. 10 ). Tracking individual cell trajectories within wounded Tg ( lyz:EGFP ) larvae revealed that neutrophils migrated with significantly reduced velocities, displacement rates and meandering indices within Irg1-depleted larvae, when compared with control larvae ( Fig. 6h–l ). Of interest, when examining migration paths of neutrophils towards wounded tissue, most neutrophils migrated ventral to somitic tissue from the caudal hematopoietic tissue (a larval hematopoietic site). Those neutrophils that migrated more medially were observed to migrate superficially in close proximity to the irg1l / mmp9 -expressing epidermis rather than through deeper somitic tissues ( Fig. 6m,n ). Together, these data suggest that, in addition to infection-driven cutaneous inflammation, Irg1l also contributes to the timely recruitment of innate immune cells to wounded tissues through regulating mmp9 expression within epidermal cells. Mouse epidermal cells upregulate IRG1 during inflammation Atopic dermatitis is an increasingly common allergic skin disease characterized by chronically relapsing cutaneous inflammation. Skin wash samples from atopic dermatitis lesions possess elevated levels of MMP9 and MMP activity, raising the possibility of a functional role for MMP9 during atopic dermatitis-associated inflammation [43] . Elevated expression of IRG1 (the mammalian homologue of zebrafish Irg1l) has only been reported in the uterine epithelium during implantation, within immune-stimulated monocytes/macrophages (where it localizes to the mitochondria) and ‘neurotoxic’ microglia [29] , [44] , [45] , [46] . We sought to explore whether IRG1 expression was also elevated within epidermal cells in a mouse model of atopic dermatitis. Using an ovalbumin-mediated epicutaneous sensitization model of atopic dermatitis, we assessed IRG1 abundance within the inflamed skin by immunohistochemistry. Strong staining for IRG1 was detected in the thickened epidermis of ovalbumin-sensitized mice (employing two different IRG1 antibodies), when compared with control (PBS-sensitized) skin biopsies ( Fig. 7a,b and Supplementary Fig. 11a,b ). Immunofluorescence revealed IRG1 was present within the mitochondria of epidermal cells ( Fig. 7c,d ). 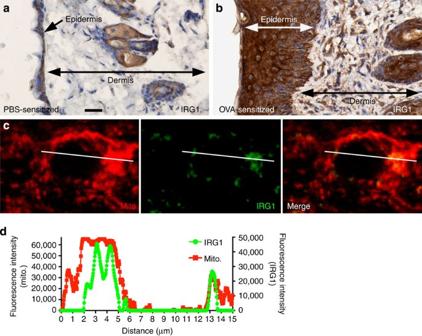Figure 7: Murine IRG1 is detected within epidermal cells in a mouse model of atopic dermatitis and localizes to the mitochondria. (a,b) Immunohistochemical staining for IRG1 within skin biopsies taken from PBS-sensitized (a) and OVA-sensitized (b) mice, respectively. (c) Immunofluorescent detection of mitochondria and IRG1 within epidermis of OVA-sensitized mouse. (d) Line fluorescence intensity measurements, for line shown inc, for Mitochondria- and IRG1-specific signals demonstrating IRG1 associates with mitochondria. Representative images fromn=4 separate PBS- and OVA-sensitized mice. Scale bars, 50 μm ina, 5 μm inc. Figure 7: Murine IRG1 is detected within epidermal cells in a mouse model of atopic dermatitis and localizes to the mitochondria. ( a , b ) Immunohistochemical staining for IRG1 within skin biopsies taken from PBS-sensitized ( a ) and OVA-sensitized ( b ) mice, respectively. ( c ) Immunofluorescent detection of mitochondria and IRG1 within epidermis of OVA-sensitized mouse. ( d ) Line fluorescence intensity measurements, for line shown in c , for Mitochondria- and IRG1-specific signals demonstrating IRG1 associates with mitochondria. Representative images from n =4 separate PBS- and OVA-sensitized mice. Scale bars, 50 μm in a , 5 μm in c . Full size image These results confirm elevated expression of IRG1 within the inflamed epidermis in a mouse model of atopic dermatitis and support a conserved role for mammalian IRG1 during cutaneous inflammation. Irg1l regulates β-oxidation-driven mROS production Beta-oxidation is the metabolic process where fatty acids are catabolized in the mitochondria to generate ATP through the OXPHOS pathway. As a by-product of OXPHOS, mitochondria produce ROS, in the form of superoxide, as electrons leak from the electron transport chain [47] . Studies have revealed that ROS can function as a signalling molecule to regulate the transcription and functional activity of various inflammatory mediators, including MMPs [14] , [15] , [48] . We have previously shown that the paralog of Irg1l, Irg1, is required within the mitochondria of activated macrophages for enhanced utilization of fatty acids that fuels mROS production [7] . We investigated whether Irg1l-dependent epidermal expression of mmp9 could be explained by a functional role for Irg1l during β-oxidation-driven mROS production. To first assess whether epidermal cells increased production of mROS following infection, we took advantage of the mitochondria-specific MitoTracker and ROS-sensitive CellROX fluorescent probes. Live imaging ROS within epidermal cells of larvae co-injected with Salmonella , MitoTracker and CellROX into the hindbrain ventricle showed that ROS was restricted to mitochondria ( Fig. 8a,b ). Quantifying overlapping CellROX/MitoTracker fluorescence signal within epidermal cells overlying the midbrain/hindbrain infection site (measured as total fluorescence intensity of colocalized signal) revealed elevated mROS production, when compared with PBS-injected controls ( Fig. 8c ). Of note, similar analysis in the presence of the mitochondrial OXPHOS inhibitor rotenone abolished this infection-driven augmentation in ROS production, confirming the ROS detected was coupled to mitochondrial OXPHOS ( Supplementary Fig. 12 ). Similar analysis within Irg1l-depleted larvae ( Fig. 8c and Supplementary Fig. 13a ) and larvae treated with an inhibitor of fatty acid β-oxidation, etomoxir ( Fig. 8d and Supplementary Fig. 13b ), demonstrated that this elevated mROS production was Irg1l- and β-oxidation-dependent. Examining mmp9 expression and macrophage recruitment within infected etomoxir-treated larvae revealed β-oxidation of fatty acids contributed to infection-responsive epidermal expression of mmp9 and macrophage recruitment ( Fig. 8e,f and Supplementary Fig. 14a,b ). Of note, etomoxir-treated larvae maintained unaltered (whole-larva) numbers of macrophages ( Supplementary Fig. 7 ). 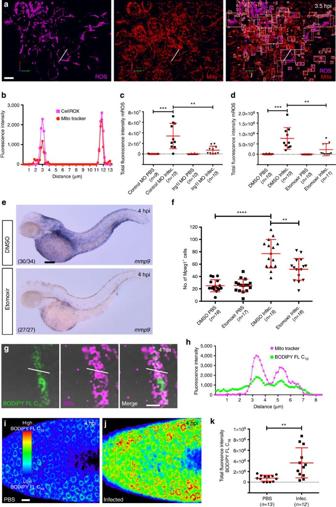Figure 8: Irg1l regulates β-oxidation-driven mROS production within epidermal cells that elevate mitochondrial uptake of fatty acids following infection. (a) Detection of mROS within epidermal cells overlying infection region. (b) Line fluorescence intensity measurements, for line shown ina, for CellROX and MitoTracker probes demonstrating overlapping peak fluorescence intensities. (c) Quantification of mROS within individual control MO-injected and Irg1l-depleted larvae following PBS control andSalmonellainjection, as detected at 3.5 hpi (mean±s.d.;n=2 separate infection experiments). (d) Quantification of mROS (as inc) within individual DMSO- and etomoxir-treated larvae injected with PBS orSalmonella(mean±s.d.;n=2 separate infection experiments). (e) Expression ofmmp9within DMSO- and etomoxir-treated larvae following infection, as detected at 4 hpi (n=2 separate infection experiments, lateral views, anterior to left). Remainder of infected DMSO-treated larvae (4/34) displayed weak epidermalmmp9expression. (f) Quantification of Mpeg1+macrophages within the midbrain/hindbrain region of DMSO- and etomoxir-treatedTg(mpeg1:EGFP) larvae at 4 hpi, following PBS orSalmonellainjections (mean±s.d.;n=2 separate infection experiments). (g) Live imaging of BODIPY FL C16and MitoTracker probe within epidermal cells overlying the midbrain/hindbrain region followingSalmonellainjection. (h) Line fluorescence intensity measurements, for line shown ing, for BODIPY FL C16and MitoTracker probes demonstrating overlapping peak fluorescence intensities. (i,j) Live imaging mitochondrial uptake of BODIPY FL C16within epidermal cells overlying the midbrain/hindbrain region following PBS (i) orSalmonella(j) injection, as detected at 4 hpi (dorsal views, anterior to left). BODIPY FL C16fluorescence intensity is displayed as a colormap, with warmer colours representing higher signal intensities. (k) Quantification of total fluorescence intensities of BODIPY FL C16within epidermal cells overlaying the midbrain/hindbrain region for individual larvae as shown iniandj(mean±s.d.;n=2 separate infection experiments). Numbers represent frequencies of larvae with displayed phenotypes. Scale bars, 10 μm ina; 100 μm ine; 5 μm ing; 20 μm ini. Statistical significance determined using a Student’st-test. **P-value <0.01; ***P-value <0.001; ****P-value <0.0001. Figure 8: Irg1l regulates β-oxidation-driven mROS production within epidermal cells that elevate mitochondrial uptake of fatty acids following infection. ( a ) Detection of mROS within epidermal cells overlying infection region. ( b ) Line fluorescence intensity measurements, for line shown in a , for CellROX and MitoTracker probes demonstrating overlapping peak fluorescence intensities. ( c ) Quantification of mROS within individual control MO-injected and Irg1l-depleted larvae following PBS control and Salmonella injection, as detected at 3.5 hpi (mean±s.d. ; n =2 separate infection experiments). ( d ) Quantification of mROS (as in c ) within individual DMSO- and etomoxir-treated larvae injected with PBS or Salmonella (mean±s.d. ; n =2 separate infection experiments). ( e ) Expression of mmp9 within DMSO- and etomoxir-treated larvae following infection, as detected at 4 hpi ( n =2 separate infection experiments, lateral views, anterior to left). Remainder of infected DMSO-treated larvae (4/34) displayed weak epidermal mmp9 expression. ( f ) Quantification of Mpeg1 + macrophages within the midbrain/hindbrain region of DMSO- and etomoxir-treated Tg ( mpeg1:EGFP ) larvae at 4 hpi, following PBS or Salmonella injections (mean±s.d. ; n =2 separate infection experiments). ( g ) Live imaging of BODIPY FL C 16 and MitoTracker probe within epidermal cells overlying the midbrain/hindbrain region following Salmonella injection. ( h ) Line fluorescence intensity measurements, for line shown in g , for BODIPY FL C 16 and MitoTracker probes demonstrating overlapping peak fluorescence intensities. ( i , j ) Live imaging mitochondrial uptake of BODIPY FL C 16 within epidermal cells overlying the midbrain/hindbrain region following PBS ( i ) or Salmonella ( j ) injection, as detected at 4 hpi (dorsal views, anterior to left). BODIPY FL C 16 fluorescence intensity is displayed as a colormap, with warmer colours representing higher signal intensities. ( k ) Quantification of total fluorescence intensities of BODIPY FL C 16 within epidermal cells overlaying the midbrain/hindbrain region for individual larvae as shown in i and j (mean±s.d. ; n =2 separate infection experiments). Numbers represent frequencies of larvae with displayed phenotypes. Scale bars, 10 μm in a ; 100 μm in e ; 5 μm in g ; 20 μm in i . Statistical significance determined using a Student’s t -test. ** P -value <0.01; *** P -value <0.001; **** P -value <0.0001. Full size image These data suggest that, in response to infection, Irg1l helps regulate β-oxidation of fatty acids within the mitochondria of epidermal cells, resulting in elevated mROS-driven mmp9 expression that contributes to macrophage recruitment. Infection enhances mitochondrial uptake of fatty acids We have previously live-imaged the subcellular trafficking of the fluorescent fatty acid analogue BODIPY FL C 16 to show that mitochondria of activated macrophages enhance their uptake of fatty acids to fuel OXPHOS-coupled mROS production [7] . We have further demonstrated that this infection-responsive process requires the activity of the zebrafish paralog of Irg1l, Irg1. Our model for Irg1l function within epidermal cells predicts similar enhanced uptake of fatty acids by the mitochondria to fuel mROS production and subsequent MMP activity. To investigate whether epidermal cells enhance their uptake of fatty acids in response to infection, we investigated the subcellular distribution of BODIPY FL C 16 within epidermal cells overlying the midbrain/hindbrain infection site. Immersion of larvae within BODIPY FL C 16 and MitoTracker probe following injection of Salmonella into the hindbrain ventricle revealed mitochondrial uptake of the fluorescent fatty acid analogue within overlying epidermal cells, as detected at 4 hpi ( Fig. 8g,h ). Of note, although BODIPY FL C 16 largely colocalized to the mitochondria, in some instances fluorescent signal was detected outside of the mitochondria, albeit in close proximity ( Fig. 8g ). This likely reflects the dynamic process of fatty acid transport to the mitochondria. Further supporting the mitochondrial uptake of BODIPY FL C 16 , mitochondrial localization within epidermal cells following infection was disrupted following treatment with etomoxir ( Supplementary Fig. 15a,b ). Etomoxir functions as an inhibitor of carnitine palmitoyltransferase-1 (ref. 49 ), a rate-limiting enzyme essential for the transport of fatty acids across the outer mitochondrial membrane. Quantifying the total fluorescence intensity of BODIPY FL C 16 within these cells showed enhanced mitochondrial uptake following infection, when compared with PBS-injected controls ( Fig. 8i–k ). These data suggest that, following infection, elevated uptake and β-oxidation of fatty acids within the mitochondria of epidermal cells fuels mROS production through an Irg1l-dependent mechanism. Enhanced mROS-driven mmp9 expression then contributes to macrophage recruitment. β-oxidation contributes to MMP production following wounding We next investigated whether similar enhanced fatty acid β-oxidation was driving Irg1l-dependent mmp9 expression and neutrophil migration within our wound-induced model of cutaneous inflammation. Similar to Irg1l-depleted larvae ( Fig. 6c,d,g ), etomoxir treatment resulted in a marked reduction in wound-induced epithelial mmp9 expression ( Fig. 9a,b ) and a significant reduction in neutrophil recruitment to tail fin wounds ( Fig. 9c ), despite maintaining unaltered whole-larvae numbers of Lyz + neutrophils ( Supplementary Fig. 10 ). We next exploited the live imaging potential of the MMPSense FAST fluorescent probe that produces fluorescence following cleavage by MMPs [50] , to live image MMP activity within tail fin wounds. Measuring the total fluorescence signal of MMPSense within a defined wound region (150 μm from the wound border), at 4 hpw, we detected wound-specific MMP activity that was both MMP9- and Irg1l-dependent ( Fig. 9d–g ). This fluorescent signal at the wound region was also significantly diminished in the presence of the pan-MMP inhibitor GM6001 and etomoxir ( Fig. 9h–k ). Zebrafish leukocytes express both mmp9 and mmp13 (refs 36 , 51 ), suggesting that they are a source of MMP activity. To confirm that the primary source of wound-induced MMP we were detecting and measuring using the MMPSense probe was epidermal, we quantified the percentage of total fluorescence intensity that was neutrophil- and macrophage-specific. Live imaging and quantification of MMPSense fluorescent signal within Tg ( lyz:EGFP ) and Tg ( mpeg1:EGFP ) larvae revealed that only 0.012±0.027% ( n=11 larvae) and 2.05±2.26% ( n=11 larvae) of the total fluorescence intensity within the wound region colocalized with Lyz + neutrophils and Mpeg1 + macrophages, respectively ( Supplementary Fig. 16 ). 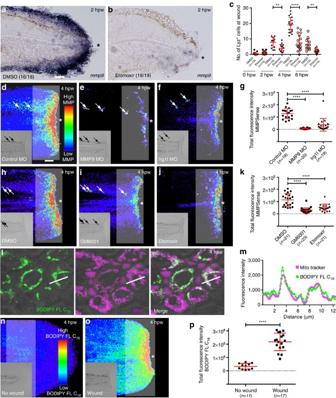Figure 9: β-oxidation and Irg1l contribute to MMP production by epidermal cells that elevate mitochondrial uptake of fatty acids following wounding. (a,b) Expression ofmmp9within wounded DMSO- and etomoxir-treated larvae, respectively, at 2 hpw (n=2 separate wounded cohorts). Remainder of wounded DMSO-treated larvae (2/18) displayed weakmmp9expression. (c) Quantification of Lyz+neutrophils within wounded DMSO- and etomoxir-treatedTg(lyz:EGFP) larvae at 0, 2, 4 and 6 hpw (mean±s.d.;n=2 separate wounded cohorts). (d–f) Live imaging MMP activity (using MMPSense 645 FAST reagent) within control MO-injected, MMP9-depleted and Irg1l-depleted wounded larvae, as detected at 4 hpw. Fluorescence intensity is displayed as a colormap, with warmer colours representing higher MMP activity. Arrows highlight pigment cell auto-fluorescence. Insets show bright field views of wounds. (g) Quantification of total fluorescence intensities of MMPSense within individual larvae as shown ind–f(mean±s.d.;n=2 separate wounded cohorts). White boxes ind–fhighlight measured region. (h–k) Live imaging and quantification of MMP activity within DMSO-, GM6001- and etomoxir-treated wounded larvae, as detected and quantified ind–g(mean±s.d.;n=2 separate wounded cohorts). (l) Live imaging BODIPY FL C16and MitoTracker probe within epidermal cells at the wound border, as detected at 4 hpw. (m) Line fluorescence intensity measurements, for line shown inl, for BODIPY FL C16and MitoTracker probes demonstrating overlapping peak fluorescence intensities. (n,o) Live imaging mitochondrial uptake of BODIPY FL C16within epidermal cells in non-wounded (n) or wounded (o) larvae, at 4 hpw. BODIPY FL C16fluorescence intensity is displayed as a colormap. (p) Quantification of total fluorescence intensities of BODIPY FL C16within epidermal cells of individual larvae as shown innando(mean±s.d.;n=2 separate wounded cohorts). Measurements taken within regions highlighted with white box. White and black asterisks mark wound border. Numbers represent frequencies of larvae with displayed phenotypes. Scale bars, 20 μm ina; 50 μm andd; 5 μm inl. Statistical significance determined using a Student’st-test. **P-value <0.01; ****P-value <0.0001. Figure 9: β-oxidation and Irg1l contribute to MMP production by epidermal cells that elevate mitochondrial uptake of fatty acids following wounding. ( a , b ) Expression of mmp9 within wounded DMSO- and etomoxir-treated larvae, respectively, at 2 hpw ( n =2 separate wounded cohorts). Remainder of wounded DMSO-treated larvae (2/18) displayed weak mmp9 expression. ( c ) Quantification of Lyz + neutrophils within wounded DMSO- and etomoxir-treated Tg ( lyz:EGFP ) larvae at 0, 2, 4 and 6 hpw (mean±s.d. ; n =2 separate wounded cohorts). ( d – f ) Live imaging MMP activity (using MMPSense 645 FAST reagent) within control MO-injected, MMP9-depleted and Irg1l-depleted wounded larvae, as detected at 4 hpw. Fluorescence intensity is displayed as a colormap, with warmer colours representing higher MMP activity. Arrows highlight pigment cell auto-fluorescence. Insets show bright field views of wounds. ( g ) Quantification of total fluorescence intensities of MMPSense within individual larvae as shown in d – f (mean±s.d. ; n =2 separate wounded cohorts). White boxes in d – f highlight measured region. ( h – k ) Live imaging and quantification of MMP activity within DMSO-, GM6001- and etomoxir-treated wounded larvae, as detected and quantified in d – g (mean±s.d. ; n =2 separate wounded cohorts). ( l ) Live imaging BODIPY FL C 16 and MitoTracker probe within epidermal cells at the wound border, as detected at 4 hpw. ( m ) Line fluorescence intensity measurements, for line shown in l , for BODIPY FL C 16 and MitoTracker probes demonstrating overlapping peak fluorescence intensities. ( n , o ) Live imaging mitochondrial uptake of BODIPY FL C 16 within epidermal cells in non-wounded ( n ) or wounded ( o ) larvae, at 4 hpw. BODIPY FL C 16 fluorescence intensity is displayed as a colormap. ( p ) Quantification of total fluorescence intensities of BODIPY FL C 16 within epidermal cells of individual larvae as shown in n and o (mean±s.d. ; n =2 separate wounded cohorts). Measurements taken within regions highlighted with white box. White and black asterisks mark wound border. Numbers represent frequencies of larvae with displayed phenotypes. Scale bars, 20 μm in a ; 50 μm and d ; 5 μm in l . Statistical significance determined using a Student’s t -test. ** P -value <0.01; **** P -value <0.0001. Full size image Wounding enhances mitochondrial uptake of fatty acids To evaluate whether the mitochondria of epidermal cells enhanced their uptake of fatty acids following wounding, similar to that observed following infection ( Fig. 8g–k ), we live-imaged the subcellular trafficking of BODIPY FL C 16 within epidermal cells following wounding. When compared with an equivalent anatomical position within the tail of non-wounded larvae, epidermal cells of wounded larvae demonstrated enhanced mitochondrial uptake of BODIPY FL C 16 ( Fig. 9l–p ) within the wound region (150 μm from the wound border). Of note, mitochondrial uptake of BODIPY FL C 16 was again inhibited following etomoxir treatment ( Supplementary Fig. 15c,d ). Similar to our infection-induced inflammation model, these results suggest that elevated uptake and β-oxidation of fatty acids within the mitochondria of epidermal cells following wounding fuels MMP production through an Irg1l-dependent mechanism. Enhanced MMP activity then contributes to the timely recruitment of neutrophils to the wound region. By exploiting the live-imaging potential of embryonic zebrafish to dissect the function of Irg1l, we have uncovered a new mechanism by which epidermal cells help direct the recruitment of leukocytes during inflammation. Using an infection-induced model of cutaneous inflammation we show that infection-responsive expression of irg1l within epidermal cells is MyD88-dependent and GC-sensitive. We predict that resident MyD88 + macrophages stimulate epidermal irg1l expression via secreted cytokines. Although strongest in epidermal cells overlying the infection site, epidermal expression of irg1l (and mmp9 ) was detected throughout the entire larvae following infection, suggesting that this macrophage-derived signal acts systemically. A previous study has shown zebrafish Cxcl8 (IL8), secreted from an unidentified cellular source at the infection site, acts systemically to trigger the rapid recruitment of leukocytes from the caudal hematopoietic tissue [52] . Investigating whether a similar systemically acting chemokine/chemokine receptor partnership operates in our model to drive epidermal expression of irg1l is a focus of future research. Of interest, infection-induced upregulation of irg1l expression within GR/Nr3c1 + oropharyngeal tissues was not suppressed following GC treatment, suggesting that the sensitivity of irg1l expression to GC-mediated suppression is tissue-specific. We provide evidence that Irg1l is necessary for the clearance of injected bacteria through helping regulate enhanced fatty acid β-oxidation to fuel mROS-driven mmp9 expression within epidermal cells, which helps direct further macrophage recruitment ( Fig. 10 ). We further reveal that a similar Irg1l-dependent immunometabolic mechanism operates within epidermal cells during wound-induced inflammation to help orchestrate the timely recruitment of neutrophils ( Fig. 10 ). In addition to uncovering a new immunometabolic function for epidermal cells during inflammation, this study represents the first whole-animal live-imaging investigation of epidermal cell metabolism during inflammation. 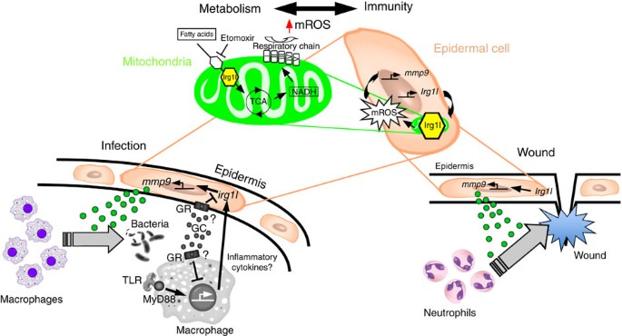Figure 10: Proposed model describing function of Irg1l within epidermal cells following infection and wounding. In response to infection, resident MyD88+macrophages signal to epidermal cells through a MyD88-dependent mechanism to induce epidermalirg1lexpression. Infection-induced epidermal expression ofirg1lis suppressed by the anti-inflammatory activity of GCs on GR+(Nr3c1+) macrophages and/or epidermal cells. Irg1l helps couple metabolism and immunity within epidermal cells through regulating fatty acid-fuelled production of mROS that contributes to epidermalmmp9expression and MMP-mediated recruitment of macrophages. In response to wounding, epidermal cells similarly couple Irg1l-dependent fatty acid-fuelled production of mROS withmmp9expression and MMP-mediated recruitment of neutrophils. Signalling components specific to infection-inducedirg1lexpression are shown in grey. TLR, toll-like receptor; GR, glucocorticoid receptor; GC, glucocorticoid; TCA, tricarboxylic acid cycle (Krebs cycle). Figure 10: Proposed model describing function of Irg1l within epidermal cells following infection and wounding. In response to infection, resident MyD88 + macrophages signal to epidermal cells through a MyD88-dependent mechanism to induce epidermal irg1l expression. Infection-induced epidermal expression of irg1l is suppressed by the anti-inflammatory activity of GCs on GR + (Nr3c1 + ) macrophages and/or epidermal cells. Irg1l helps couple metabolism and immunity within epidermal cells through regulating fatty acid-fuelled production of mROS that contributes to epidermal mmp9 expression and MMP-mediated recruitment of macrophages. In response to wounding, epidermal cells similarly couple Irg1l-dependent fatty acid-fuelled production of mROS with mmp9 expression and MMP-mediated recruitment of neutrophils. Signalling components specific to infection-induced irg1l expression are shown in grey. TLR, toll-like receptor; GR, glucocorticoid receptor; GC, glucocorticoid; TCA, tricarboxylic acid cycle (Krebs cycle). Full size image Zebrafish possess co-orthologues for IRG1 ( irg1 and irg1l ). Our previous study has established a role for zebrafish Irg1 in coupling metabolism with immune cell function within macrophages [7] . We showed that irg1 was specifically expressed within immune-stimulated macrophages where the encoded enzyme was required for enhanced β-oxidation of fatty acids to fuel OXPHOS-coupled mROS production. Here we demonstrate a similar role for Irg1l during enhanced utilization of fatty acids to fuel mROS production within epidermal cells during infection- and wound-induced inflammation. To date, mammalian IRG1 expression has been reported in activated macrophages, neurotoxic microglia and within the uterine epithelium [44] , [46] , [53] . IRG1 has been shown to localize to the mitochondria using fluorescent fusion proteins and cell fractionation experiments [45] . Functional experiments further support a mitochondrial association [7] , [54] . Employing a mouse model of atopic dermatitis and antibodies against human IRG1, we have shown elevated levels of IRG1, as detected by immunofluorescence, within the inflamed skin of ovalbumin-sensitized mice, where it associates with the mitochondria of keratinocytes. Our model predicts IRG1 is required for enhanced β-oxidation of fatty acids within keratinocytes during inflammation. In all eukaryotic organisms, β-oxidation occurs in mitochondria and peroxisomes [55] . It is emerging that, in response to inflammatory stress, mitochondria are highly dynamic and can form intimate physical interactions with other organelles (including peroxisomes and mitochondrial-associated endoplasmic reticulum membranes) [56] . These interactions are believed to form signalling scaffolds that help coordinate immune cell function. Identifying how IRG1 associates with the mitochondria in our mouse dermatitis model, by generating mouse-specific IRG1 antibodies and performing immunogold labelling/transmission electron microscopy, is a focus of future research. Our results support a conserved immunometabolic role for IRG1 within mammalian epidermal cells during cutaneous inflammation and suggest that the function of mammalian IRG1 is subfunctionally partitioned between Irg1 and Irg1l in zebrafish. Subfunctional partitioning is common with duplicated genes resulting from the pre-teleost genome duplication. Occupying separate loci, duplicate genes are independently mutable and can acquire mutations within regulatory elements that help direct tissue-specific expression. This can lead to paralogs with tissue-specific functions that cumulatively recapitulate that of the ancestral gene [57] . Unlike ray-finned fish and reptiles, mammals possess one IRG1 orthologue ( http://www.ensembl.org/Danio_rerio/Gene/Compara_Tree?g=ENSDARG00000069844;r=9:22866973-22871390 ), suggesting that degenerative mutations in coding and/or regulatory regions (nonfunctionalization) have contributed to the loss of one of the gene duplicates in this lineage, a fate that accounts for most duplicated genes [58] . Our model predicts that, during cutaneous inflammation, elevated β-oxidation of fatty acids within epidermal cells contributes to the recruitment of leukocytes through mROS-driven augmentation of mmp9 expression. MMPs are well-recognized mediators of inflammation and innate immune cell activity [59] . By directly modulating chemokine gradients and degrading ECM components, MMPs shape the outcome of inflammation by helping direct the recruitment of innate immune effector cells (including neutrophils and monocytes/macrophages) to sites of infection or injury [59] . During cutaneous inflammation, keratinocytes are a major source of MMP activity (including that provided by MMP-9) that, in addition to regulating re-epithelialization, are believed to contribute to leukocyte recruitment [13] , [59] . Supporting a connection between mitochondrial redox signalling and MMP activity, evidence suggests that mROS-sensitive signalling pathways direct both the expression and activity of MMP family members [14] . Furthermore, heat shock-induced MMP-9 expression within a human keratinocyte cell line is, in part, regulated by mROS [60] , and TNF-α-stimulated human keratinocytes enhance production of MMP-9 through a ROS/NF-κB-dependent mechanism [15] . Our study reveals the contribution of mROS-driven MMP activity towards leukocyte recruitment is fuelled by metabolic reprogramming in keratinocytes towards elevated fatty acid β-oxidation. Supporting a connection between elevated β-oxidation and the inflammatory response during cutaneous inflammation, the expression of enzymes associated with fatty acid oxidation are elevated within the skin of patients with the inflammatory dermatosis psoriasis [61] , [62] . It has also been suggested that epidermal fatty acid-binding protein contributes to the pathogenesis of psoriasis through activation of the NF-κB signalling pathway [63] , a powerful transcriptional regulator of pro-inflammatory genes. Furthermore, etomoxir-mediated β-oxidation inhibition is beneficial in the treatment of psoriasis [64] . We provide a mechanistic link connecting enhanced fatty acid β-oxidation within epidermal cells to their immune function that acts to direct leukocyte recruitment. The precise mechanism through which Irg1l/IRG1 participates during β-oxidation-fuelled augmentation of mROS is the focus of future work. Metabolic reprogramming as a strategy to regulate the immune response is known to operate within immune cells [3] , [4] . To our knowledge, this study describes the first example of metabolic reprogramming being employed within a non-immune cell type to help shape its contribution to the immune response. Pharmacologic targeting of this metabolic–immunological interface within keratinocytes may prove efficacious in treating inflammatory dermatoses. Zebrafish maintenance Zebrafish ( Danio rerio ) embryos were obtained from natural spawnings and raised at 28 °C in E3 Medium supplemented with 0.003% phenylthiourea (PTU) to inhibit pigmentation. The Tg ( mpeg1:Gal4-VP16 ) gl24 ; Tg ( UAS-E1b:Kaede ) s1999t (herein referred to as Tg ( mpeg1:Gal4/UAS:Kaede )), Tg ( mpeg1:EGFP ) gl22 , Tg ( mpeg1:mCherry ) gl23 , Tg ( lyz:EGFP ) NZ117 and Tg ( ef1- α : DsRED2 ) transgenic reporter lines were used in this study. Research was conducted with approval from the University of Auckland Animal Ethics Committee. Mice Six to 8-week-old female C57BL/6 mice were bred and housed in the Animal Resource Unit, Faculty of Medical and Health Sciences, University of Auckland, Auckland, New Zealand. The mice were kept in an air-conditioned room with controlled humidity, temperature and a 12 h light/dark cycle. All experiments were conducted under a protocol approved by the University of Auckland Animal Ethics Committee. Live bacterial and LPS injection of zebrafish larvae Zebafish larvae were injected with non-fluorescent wild-type or GFP-expressing S. enterica serovar Typhimurium into the hindbrain ventricle as previously described [31] . In brief, anaesthetized 2 dpf larvae were mounted in 3% methyl cellulose (in E3 media) and injected with 1 nl of bacterial injection preparation (~\n600 cfu/nl in filter-sterilized PBS) into the hindbrain ventricle. Immediately before and after injecting a cohort of larvae, an injection bolus was injected into filter-sterilized PBS (in duplicate) that was plated at 1:10 and 1:100 dilutions to quantify and validate infection dose. LPS ( E. coli K12, InvivoGen) was similarly injected (0.8 mg ml −1 , 1 nl), as previously described [7] . Microarray and analysis Total RNA was extracted from dissected trunks of infected and PBS control-injected larvae at 2 dpi (injected at 2 dpf) using TRIzol reagent (Invitrogen) and purified using Qiagen RNeasy columns as per the manufacturer’s instructions. Hybridization to Affymetrix GeneChip Zebrafish Genome arrays and data acquisition were performed at the Centre for Genomics and Proteomics, School of Biological Sciences, University of Auckland. Data were normalized using the RMA method and statistical analysis of differential expression between control and infected larval zebrafish trunks was performed using linear models (LIMMA). Whole-mount in situ hybridization WMISH was performed using digoxigenin and fluorescein-labelled riboprobes (Roche) and BM purple (Roche) colour precipitation or Tyramide Signal Amplification (Invitrogen) for fluorescent WMISH analysis, as previously described [31] , [65] . RT–PCR Total RNA was extracted from embryos and larvae using TRIzol reagent (Invitrogen) as per the manufacturer’s instructions. Superscript III reverse transcriptase (Invitrogen)-generated cDNAs were used to produce gene-specific amplicons using primer pairs designed to span at least 1 intron to control for contaminating genomic DNA. To assess Irg1l and MMP9 MO specificities the following (forward/reverse) primer pairs were used, 5′-TCCAGATCCTGACCACAAC-3′/5′-TTATTGCAGTTGGGCAAGC-3′ and 5′-CTGATCTGATCTGAGCACTTGC-3′/5′-GCTGACGGACAAATATGCCTAAC-3′ respectively. Primers to ef1- α (5′-AAGGAGAAGATCGACCGTCG-3′ and 5′-TGATTGAGGGAAATTCACTTGG-3′) were used as an internal control. To generate irg1l- , krt4- and mmp9 -targeting riboprobes the following primer pairs were used: irg1l , 5′-TCCAGATCCTGACCACAAC-3′ and 5′-TTATTGCAGTTGGGCAAGC-3′; krt4 , 5′-ATGGGCTTTGTTGCGGCTCCTATC-3′ and 5′-TGAGTCGTAAGAAGGTTCAGAAGGG-3′; mmp9 , 5′-CGACTCAAGATGAGACTTGGAG-3′ and 5′-GCTGACGGACAAATATGCCTAAC-3′. Riboprobes to detect myd88 were as previously described [18] . MO injection MOs (Gene Tools, Philomath, OR, USA) were resuspended in sterile water and injected in 1 × Danieau’s solution. Efficacious doses for all MOs were determined empirically. RT–PCR was used to determine MO specificity where splice-blocking MOs were used. Sequences of MOs (and doses) are as follows: control MO, 5′-CCTCTTACCTCAGTTACAATTTATA-3′ (1.5 pmole); Nr3c1 MO (splice-blocking), 5′-GCCAGAGATATATGGAATACCTTCA-3′ (0.5 pmole) [7] ; Irg1l MO (splice-blocking), 5′-AACACATTAGGCAGTACTTACTGCT-3′ (1.5 pmole); Nr5a1a MO (translation-blocking), 5′-AATCCTCATCTGCTCTGAAGTC-3′ (0.5 pmole) [37] ; Irf8 MO (splice-blocking), 5′-AATGTTTCGCTTACTTTGAAAATGG-3′ (1.5 pmole) [33] ; MyD88 MO (splice-blocking), 5′-GGTTAAACACTGACCCTGTGGATC-3′ (1.0 pmole) [7] ; Gcsrf MO (splice-blocking), 5′-ATTCAAGCACATACTCACTTCCATT-3′ (0.5 pmole) [31] ; Spi1 MO (translation-blocking), 5′-GATATACTGATACTCCATTGGTGGT-3′ (1.0 pmole) [66] ; MMP9 MO (splice-blocking), 5′-ATACAAAATACTCGACTCACCTGCT-3′ (0.25 pmole). Confocal imaging Live embryos and larvae were mounted for confocal imaging, as previously described [67] . All live confocal imaging was performed on an Olympus FV1000 FluoView laser scanning confocal microscope equipped with an incubation chamber. Confocal imaging of fluorescent WMISH was performed using a Nikon C1 Eclipse confocal microscope. Images collected by confocal microscopy were processed and analysed using Volocity 6.1.1 (Perkin Elmer). To detect ROS production and mitochondria, the CellROX Deep Red Reagent (Invitrogen C10422, 1 nl at 50 μM, absorption/emission maxima of ~\n644/665 nm) and MitoTracker Red CMXRos (Invitrogen M7512, 1 nl at 20 μM, absorption/emission maxima of ~\n579/599 nm) fluorescent dyes were injected into the hindbrain ventricle, respectively. To live image BODIPY FL C 16 and mitochondria larvae were immersed in 50 μM BODIPY FL C 16 (Invitrogen, D-3821, imaged using absorption/emission maxima as used to detect Alexa Fluor 488 (~\n495/519 nm)) and 1 μM MitoTracker Deep Red FM (Invitrogen M22426, absorption/emission maxima of ~\n644/665 nm), respectively, for 2 h immediately following infection or tail transection, washed for 30 min in PTU-treated E3 medium before mounting and imaging. To live image MMP activity, larvae were immersed in 40 μM MMPSense 645 FAST (Perkin Elmer, NEV10100, absorption/emission maxima of ~\n649/666 nm) for 2 h immediately following tail transection, washed for 30 min in PTU-treated E3 medium before mounting and imaging. When quantifying mROS, MMP activity and BODIPY FL C 16 uptake using fluorescence intensity measurements, conservative laser excitation settings were used to ensure that we did not create/measure a saturated fluorescence signal. See Supplementary Methods for detailed descriptions of confocal imaging/analysis when used for neutrophil tracking and quantification of macrophage numbers at infection site, mROS production, BODIPY FL C 16 fluorescence and MMPSense FAST fluorescence. Chemical treatments The following chemical agonists and antagonists were used. No abnormal development or toxicity was observed for all compounds used at the indicated working concentrations and routes of delivery. The GR antagonist RU-486 (Sigma, M8046) was delivered by immersion (2 h pre-treatment before infection, 250 μM 1% DMSO). The β-oxidation inhibitor etomoxir (Sigma, E1905) was delivered by immersion (1–2 h pre-treatment before infection or wounding, 100 μM for infection and 10 μM for wounding experiments, 1% DMSO). The OXPHOS inhibitor rotenone (Sigma, R8875) was delivered by immersion (1–2 h pre-treatment before infection, 1 μM 1% DMSO). The MMP inhibitor GM6001 (Sigma, M5939) was delivered by immersion (1–2 h pre-treatment before wounding, 200 μM 1% DMSO). The GR agonists dexamethasone (Sigma), prednisolone (Sigma) and hydrocortisone (Sigma) were injected into the hindbrain ventricle (1 nl at 0.67 mg ml −1 ) with PBS or Salmonella . Anti-inflammatory activities of dexamethasone, prednisolone and hydrocortisone (delivered by immersion at ~\n5 μM, 1% DMSO) were assessed by their ability to inhibit neutrophil migration using an acute tail-wounding assay with 3 dpf Tg ( lyz:EGFP ) larvae. Quantitative PCR qPCR was performed with Platinum SYBR Green qPCR SuperMix-UDG with ROX (Invitrogen) using an ABI PRISM 7900HT Fast sequence detection system (Applied Biosystems) as previously described [68] . Gene-specific oligonucleotides were designed using Primer Express software to detect irg1l (5′-CACTAGATGTGGCAGAGCGT-3′ and 5′-CCCAACTCCAATGCTGTCTA-3′), mmp9 (5′-TGGGCACCTGCTCGTTGA-3′ and 5′-TTGGAGATGACCGCCTGC-3′) and ef1- α (5′-TGCCTTCGTCCCAATTTCAG-3′ and 5′-TACCCTCCTTGCGCTCAATC-3′). All reactions were performed in biological triplicate and technical quadruplicate and a melting curve analysis carried out to confirm reaction specificity. Analysis used the comparative CT method with ef1- α as an internal control. Individual CFU counts Individual CFU counts of larvae infected with Sal-GFP was performed as previously described [69] . Larval homogenates were plated in a dilution series on LB agar plates supplemented with 25 μg ml −1 kanamycin. Acute tail wounding An acute tail fin wound was generated by transecting the tail fin of anaesthetized 2 dpf larvae using a sterile scalpel. Care was taken to transect tails at exactly the same anatomic location (posterior-most edge of notochord). Flow cytometry Flow cytometry was performed as previously described [18] . In brief, larvae were rinsed in calcium-free Ringer’s solution for 15 min before removal of yolks by repeated passage through a 200 μl pipette tip. Larvae were then digested in 0.25% trypsin-EDTA (Gibco) for 2 h at 28.5 °C with manual dissociation every 10 min. The digestion was inhibited by the addition of CaCl 2 to a concentration of 1 mM and 5% FBS. The dissociated cells were centrifuged for 5 min at 3,000 r.p.m. before resuspension in ice-cold 0.9 × PBS, 5% FBS. Cells were passed several times through 40-μm cell strainers (BD Falcon) before sorting. Flow cytometry was performed using a Becton Dickinson LSRII flow cytometer. Immunofluorescence and immunohistochemistry Immunohistochemical staining of paraffin sections was performed using the Vectastain elite ABC kit (Vector Laboratories, PK-6100) as per the manufacturer’s instructions. Immunofluorescence was carried out as previously described [18] . Primary and secondary antibody combinations used were the following: chicken anti-GFP (1:500/Abcam, ab13970) with goat anti-chicken Alexa Fluor 488 (1:500/Invitrogen); rabbit anti-Kaede (1:500/MBL, PM012) with goat anti-rabbit Alexa Fluor 633 or goat anti-rabbit Alexa Fluor 488 (1:500/Invitrogen); rabbit anti-Human GR (P-20) (1:75/Santa Cruz Biotechnology Inc., sc-1002) with goat anti-rabbit Alexa Fluor 546 (1:500/Invitrogen); rabbit anti-human IRG1 (1:300/N-20, sc-84191 and C-18, sc-84189, Santa Cruz Biotech.) with goat anti-rabbit Alexa Fluor 488 (1:500/Invitrogen) or biotinylated horse anti-rabbit IgG; mouse anti-mitochondria antibody (1:500/Abcam, ab3298) with goat anti-mouse Alexa Fluor 568 (1:500/Invitrogen). Ovalbumin-mediated epicutaneous sensitization model of AD The protocol for inducing atopic dermatitis was as previously described [70] . In brief, mice were shaved, and the dorsal skin tape-stripped six times under anaesthesia. Ovalbumin (100 μg in 100 μl of PBS) or PBS (as a negative control) was placed on a patch of gauze (1 × 1 cm), which was secured to the skin site with a transparent bio-occlusive dressing for a 1-week period and then removed. Each mouse received a total of three 1-week exposures to a patch separated by 2-week patch-free intervals. Mice were monitored daily to ensure that patches remained in place throughout the sensitization period. Mice were killed 24 h after removal of the third patch and skin tissue samples were collected. Skin tissues were fixed in 10% formalin, embedded into paraffin and sectioned. Statistical analysis Statistical analyses were performed using Prism 5.0 (GraphPad Software, Inc.). Statistical significance was assessed using unpaired, two-tailed t -tests and all data presented in scatter plots show means with s.d. P values <0.05 were considered statistically significant. Accession codes : Microarray data used in this study have been deposited in the Gene Expression Omnibus, accession number GSE56365 . How to cite this article: Hall, C. J. et al. Epidermal cells help coordinate leukocyte migration during inflammation through fatty acid-fuelled matrix metalloproteinase production. Nat. Commun. 5:3880 doi: 10.1038/ncomms4880 (2014).